ROW1 maintains quiescent centre identity by confiningWOX5expression to specific cells The quiescent centre (QC) in the Arabidopsis root apical meristem is essential for stem cell organization. Here we show that the loss of REPRESSOR OF WUSCHEL1 (ROW1), a PHD domain-containing protein, leads to QC failure, defects in cell differentiation and ectopic expression of WUSCHEL-RELATED HOMEOBOX 5 ( WOX5 ) in cells that normally express ROW1 . The wox5-1/row1-3 double mutants show similar phenotypes to wox5-1 indicating that WOX5 is epistatic to ROW1. ROW1 specifically binds trimethylated histone H3 lysine 4 (H3K4me3) in the WOX5 promoter region to repress its transcription. QC expression of ROW1 results in a wox5-1 -like phenotype with undetectable WOX5 transcripts. We propose that ROW1 is essential for QC maintenance and for stem cell niche development through the repression of WOX5 in the proximal meristem. A plant seedling typically starts out with two meristems, which are situated at the tip of the shoot and the root [1] . The organizing centre (OC) and the quiescent centre (QC) play essential roles in maintaining stem cell populations within shoot and root meristems, respectively [2] , [3] . OC-specific WUS transcription is required for stem cell homeostasis in the shoot apical meristem (SAM) [4] , [5] . CLAVATA 3 (CLV3), a small peptide specifically expressed in the central zone immediately above the OC, represses WUS expression outside of the OC by binding to another small peptide CLV1 (ref. 6 ). Activation of CLV1 and related receptor kinases mediates the repression of WUS transcription through a signalling cascade that is not well understood [7] , [8] . On the other hand, OC-expressed WUS was found to migrate into the central zone to activate CLV3 transcription in a feedback loop [9] that maintains the number of stem cells in the SAM. Likewise, the stem cell population in the root apical meristem is maintained by confining the expression of WUSCHEL-RELATED HOMEOBOX 5 ( WOX5 ), a homeobox transcription factor [10] , [11] to the QC. The root stem cell niche is positioned in the apical–basal direction along an auxin gradient, which is produced by the polar localization of PIN-FORMED proteins [12] . Auxin regulates distal meristem (DM) cell differentiation by acting on WOX5 (ref. 13 ). AUXIN RESISTANT 3 (AXR3), a member of the AUX/IAA family, is required for auxin signalling through the auxin response factors ARF10 and ARF16 (refs 13 , 14 ). Recent work revealed that the WOX5–AXR3 feedback circuit is essential for the auxin-mediated DM differentiation in the Arabidopsis root [15] . To date, the mechanisms of QC-specific WOX5 expression, QC identity maintenance and proximal meristem (PM) differentiation remain largely unknown. The first discovered plant homeodomain (PHD)-containing protein with a canonical Cys4-His-Cys3 zinc finger motif was HAT3.1 (ref. 16 ), which regulates nuclear processes involving chromatin covalent modifications, especially histone H3 lysine 4 (H3K4) methylation [17] , [18] . Trimethylated H3K4 (H3K4me3) is proposed to regulate gene expression through its recognition by transcriptional activators [19] , [20] . Previous studies revealed that certain PHD domain-containing proteins bind to H3K4me3 to regulate target gene transcription via histone acetyl transferase activities or histone deacetylase chromatin-modifying complexes [20] , [21] , [22] . REPRESSOR OF WUS1 (ROW1) is a PHD-containing protein [23] with two tandem BRCA1 C-terminal domains and a RING domain [24] . The BRCA1 C-terminal domains of ROW1 are important for phosphorylation-dependent protein–protein interactions [25] , and the RING domain is required for DNA repair [26] . Mutations in ROW1 (formerly called BARD1 (ref. 23 )) cause severe SAM defects in Arabidopsis by releasing WUS expression from its normal confinement in the OC to the outermost cell layers [24] . In this study, we show that ROW1 is required to maintain QC identity and stem cell niche development. We propose that it functions by suppressing WOX5 expression in the PM of Arabidopsis root. We believe that it is the first key repressor that maintains both root apical meristem and SAM structures by interacting with WUS and WOX5 independently. Root phenotypes of the Arabidopsis row1-3 mutant Here we observed severe root architecture defects, including extremely short roots ( Fig. 1a ) and loss of gravitropic response ( Fig. 1b ) in the row1-3 knockout mutant. Median longitudinal semi-thin sections showed no obvious QC identity, no distal root meristem (DSC) structure and no starch granules that indicates a defect in columella cell differentiation in the mutant (compare the wild type shown on the left of Fig. 1c to the mutant on the right). Sections prepared from the maturation zone, however, displayed a drastic difference in cell length between the two seedlings ( Fig. 1d ). Interestingly, the loss of gravitropism in row1-3 was independent of auxin signalling, because both mutant and wild-type seedlings showed similar expression patterns of the synthetic auxin-responsive promoter reporter DR5::GFP after gravistimulation ( Supplementary Fig. 1 ). In row1-3 roots, root hair cells emerged very close to the root tip, indicating that its PM is defective and largely consumed ( Fig. 1e , with a wild-type root shown on the left and row1-3 on the right). The root tips of row1-3 are devoid of starch granules as evidenced by lack of staining with Lugol’s solution ( Fig. 1f ), indicating a complete repression of columella cell differentiation. Furthermore, a green fluorescent protein (GFP)-fusion reporter of SCARECROW (SCR), normally expressed specifically in the QC and the entire endodermis ( Fig. 1g , left) [27] , was absent from the QC in row1-3 mutants ( Fig. 1g , right), indicating the loss of the QC identity. Meanwhile, the GFP-enhancer trap line J0571, specifically expressed in the QC and cortex/endodermis in wild type ( Fig. 1h , left) [27] , [28] , was also absent from row1-3 ( Fig. 1h , right). Both these experiments indicated the loss of the QC identity in the mutant. 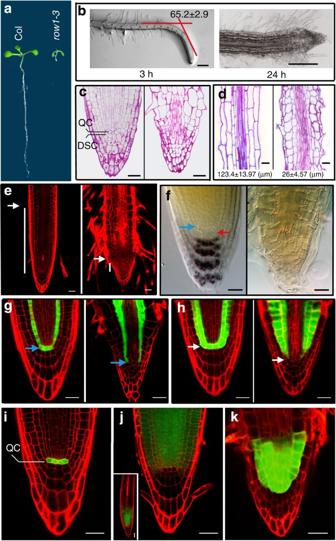Figure 1: Phenotypic and expression pattern analysis inrow1-3roots. (a) A 2-week-old wild-typeArabidopsisseedling (Col) showed normal root length (left), whereas arow1-3root (right) did not elongate. (b) Gravitropic responses in wild-type (left) androw1-3(right) roots. Degrees of bending (mean±s.e.) were calculated from 10 independent main roots of each type. (c) Median longitudinal semi-thin sections of 7-day-old wild-type (left) androw1-3(right) root tips stained with periodic acid–Schiff solution. (d) Cell length measurements from maturation zone in wild-type (wt) androw1-3roots. Root tips from 7-day-old seedlings were used for semi-thin section preparations; cell lengths (mean±s.e. in μm) were obtained from three seedlings of each type. (e) 7-day-old root tips of wild type (left) androw1-3(right). White bars indicate the size of PM regions. (f) Wild-type root tip accumulated starch granules in columella cells (left), whereas no starch granule was observed inrow1-3root tips (right). Starch granules were stained with the Lugol’s solution and seen as aggregated black spots. Blue arrow, QC position; red arrow, DSC layer. (g) SCR::GFP expression showing normal QC identity (blue bars) in the wild-type (left) and a defective QC position inrow1-3roots (right). (h) Expression pattern analysis of the GFP-enhancer trap line J0571 that show normal QC identity in the wild type (left) with a defective QC inrow1-3roots (right). (i) WOX5::GFP signals were detected specifically in the QC in wild-type seedlings. (j) ROW1::GFP signals were detected above, but not in, the QC position in wild-type seedlings. Inset, a lower-magnification micrograph shows the whole root tip. (k) WOX5::GFP signals were detected in cells above the normal QC position inrow1-3root. Scale bars, 20 μm in this figure. Figure 1: Phenotypic and expression pattern analysis in row1-3 roots. ( a ) A 2-week-old wild-type Arabidopsis seedling (Col) showed normal root length (left), whereas a row1-3 root (right) did not elongate. ( b ) Gravitropic responses in wild-type (left) and row1-3 (right) roots. Degrees of bending (mean±s.e.) were calculated from 10 independent main roots of each type. ( c ) Median longitudinal semi-thin sections of 7-day-old wild-type (left) and row1-3 (right) root tips stained with periodic acid–Schiff solution. ( d ) Cell length measurements from maturation zone in wild-type (wt) and row1-3 roots. Root tips from 7-day-old seedlings were used for semi-thin section preparations; cell lengths (mean±s.e. in μm) were obtained from three seedlings of each type. ( e ) 7-day-old root tips of wild type (left) and row1-3 (right). White bars indicate the size of PM regions. ( f ) Wild-type root tip accumulated starch granules in columella cells (left), whereas no starch granule was observed in row1-3 root tips (right). Starch granules were stained with the Lugol’s solution and seen as aggregated black spots. Blue arrow, QC position; red arrow, DSC layer. ( g ) SCR::GFP expression showing normal QC identity (blue bars) in the wild-type (left) and a defective QC position in row1-3 roots (right). ( h ) Expression pattern analysis of the GFP-enhancer trap line J0571 that show normal QC identity in the wild type (left) with a defective QC in row1-3 roots (right). ( i ) WOX5::GFP signals were detected specifically in the QC in wild-type seedlings. ( j ) ROW1::GFP signals were detected above, but not in, the QC position in wild-type seedlings. Inset, a lower-magnification micrograph shows the whole root tip. ( k ) WOX5::GFP signals were detected in cells above the normal QC position in row1-3 root. Scale bars, 20 μm in this figure. Full size image Identification of WOX5 as a target of ROW1 in roots Because WUS is not expressed in the Arabidopsis root ( Supplementary Fig. 2a ) [29] , we analysed the WOX transcription factor gene family for possible ROW1 targets ( Supplementary Fig. 3 ). Quantitative reverse transcription-PCR (qRT–PCR) analysis identified WOX5 as the most significantly (<0.001) upregulated WOX gene in row1-3 roots ( Supplementary Fig. 2b ). In contrast, wild-type levels of ROW1 transcript were found in the wox5-1 -knockout mutant ( Supplementary Fig. 2c ). Further experiments, in corroboration with previous reports [30] , [31] , confirmed the exclusive expression of WOX5 in the QC of wild-type roots ( Fig. 1i ), while ROW1 is expressed in the PM above the QC ( Fig. 1j ). In row1-3 , however, the WOX5 expression zone is expanded into the multiple PM cell layers ( Fig. 1k ), suggesting that WOX5 may be a target of ROW1. The row1-3 root phenotype is complemented in wox5-1 Homozygous wox5-1/row1-3 double-mutant seedlings showed substantial root elongation ( Figs 1a and 2a ) and PM restoration ( Fig. 2c ), compared with the row1-3 mutant. The gravitropic curvature of wox5-1/row1-3 is similar to wox5-1 ( Fig. 2b ). QC identity and columella cell differentiation are both restored in the double mutant as indicated by SCR::GFP signal ( Fig. 2d ), J0571 marker ( Fig. 2e ) and Lugol’s solution staining ( Fig. 2f ). Similar to wox5-1 , substantial amounts of starch granules accumulated in the DSC layer in wox5-1/row1-3 roots ( Fig. 2f ), suggesting that these cells underwent premature differentiation. 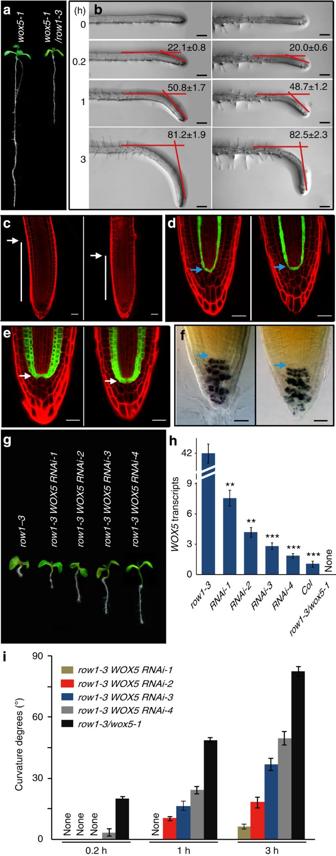Figure 2: Complementation of therow1-3phenotype in thewox5-1/row1-3double mutant and inrow1-3 WOX5RNAi lines. (a) Comparisons of root lengths at the 2-week-old stage. Thewox5-1seedling has a root length similar to that of wild type; thewox5-1/row1-3double-mutant root was significantly elongated as compared with that of therow1-3single mutant (Fig. 1a). (b) Faster gravitropic responses were observed in roots of bothwox5-1(left) andwox5-1/row1-3(right). Degrees of bending (mean±s.e.) were obtained from 10 seedlings. (c) 7-day-old root tips ofwox5-1(left) andwox5-1/row1-3double mutant (right). White bars indicate the size of PM regions. (d) SCR::GFP expression indicating QC identity (blue arrow) inwox5-1(left) and also in thewox5-1/row1-3double mutant (right). (e) The GFP-enhancer trap line J0571 showing QC identity (white arrow) both inwox5-1(left) and in thewox5-1/row1-3double mutant (right). (f) Root tips of thewox5-1/row1-3double mutant (right) accumulated starch granules not only in columella cells but also in the DSC layer, identical towox5-1(left). (g) Photographs of 7-day-oldrow1-3 WOX5 RNAi-1,-2,-3and-4in comparisons withrow1-3and thewox5-1/row1-3double mutant. (h) qRT–PCR analysis ofWOX5mRNA levels inrow1-3,row1-3 WOX5RNAi lines, wild-type andwox5-1/row1-3roots, Error bars represent s.e. from three biological replicates. **, *** denotesP<0.01 orP<0.001, compared with therow1-3, respectively. (i) Comparisons of gravitropic responses of variousrow1-3 WOX5RNAi lines andwox5-1/row1-3. Degrees of bending (mean±s.e.) were calculated from 10 seedlings. Scale bars, 100 μm in (b) and 20 μm in (c–f). Figure 2: Complementation of the row1-3 phenotype in the wox5-1 / row1-3 double mutant and in row1-3 WOX5 RNAi lines. ( a ) Comparisons of root lengths at the 2-week-old stage. The wox5-1 seedling has a root length similar to that of wild type; the wox5-1 / row1-3 double-mutant root was significantly elongated as compared with that of the row1-3 single mutant ( Fig. 1a ). ( b ) Faster gravitropic responses were observed in roots of both wox5-1 (left) and wox5-1/row1-3 (right). Degrees of bending (mean±s.e.) were obtained from 10 seedlings. ( c ) 7-day-old root tips of wox5-1 (left) and wox5-1/row1-3 double mutant (right). White bars indicate the size of PM regions. ( d ) SCR::GFP expression indicating QC identity (blue arrow) in wox5-1 (left) and also in the wox5-1/row1-3 double mutant (right). ( e ) The GFP-enhancer trap line J0571 showing QC identity (white arrow) both in wox5-1 (left) and in the wox5-1/row1-3 double mutant (right). ( f ) Root tips of the wox5-1/row1-3 double mutant (right) accumulated starch granules not only in columella cells but also in the DSC layer, identical to wox5-1 (left). ( g ) Photographs of 7-day-old row1-3 WOX5 RNAi-1 , -2 , -3 and -4 in comparisons with row1-3 and the wox5-1/row1-3 double mutant. ( h ) qRT–PCR analysis of WOX5 mRNA levels in row1-3 , row1-3 WOX5 RNAi lines, wild-type and wox5-1/row1-3 roots, Error bars represent s.e. from three biological replicates. **, *** denotes P <0.01 or P <0.001, compared with the row1-3 , respectively. ( i ) Comparisons of gravitropic responses of various row1-3 WOX5 RNAi lines and wox5-1/row1-3 . Degrees of bending (mean±s.e.) were calculated from 10 seedlings. Scale bars, 100 μm in ( b ) and 20 μm in ( c – f ). Full size image The row1-3 root phenotype is restored in WOX5 RNAi lines To examine more closely whether WOX5 is a direct target of ROW1 function and that the defective root phenotype of row1-3 is caused by ectopic WOX5 expression, we used RNA interference (RNAi) to knockdown WOX5 expression in the row1-3 mutant. A series of RNAi lines, named row1-3 WOX5 RNAi-1 , -2 , -3 and -4 , were obtained based on their different root lengths, which correlated inversely with WOX5 expression ( Fig. 2g,h ). Cells in the maturation zone of the RNAi lines were progressively longer than those in row1-3 ( Supplementary Fig. 4 ). The strongest RNAi line showed gravitropic responses close to the wox5-1/row1-3 double mutant ( Fig. 2i ). ROW1 binds to H3K4me3 located at WOX5 promoter region Next we studied the possible molecular interaction between ROW1 and WOX5 using various fragments of the WOX5 promoter depicted in Fig. 3a . The CAAT and TATA boxes were found –73 and –32 bp, respectively, upstream of the WOX5 transcription initiation site as predicted by PlantCARE ( http://bioinformatics.psb.ugent.be/webtools/plantcare/html/ ). We used a ROW1-specific polyclonal antibody generated against its C-terminal domain [24] for chromatin immunoprecipitation (ChIP) analysis and found that this antibody specifically pulled down the proximal WOX5 promoter region (fragments P3 and P4; Fig. 3b ). In vitro -expressed and -purified His-ROW1-PHD specifically immunoprecipitated H3K4me3 but not H3K4me1 or H3K4me2 ( Fig. 3c ). This construct was also unable to pull down H3K9me3 and H3K27me3 ( Supplementary Fig. 5 ). Theoretical nucleosome positioning analysis [32] revealed that the proximal WOX5 promoter region corresponding to P3 and P4 is likely packed into nucleosomes ( Fig. 3d ). The WOX5 promoter with its P3 or P4 fragment deleted lost the ability to restore the wox5-1 root phenotype ( Supplementary Fig. 6a ). At the molecular level, deletion of either one of the two fragments resulted in a non-functional promoter with no GFP expression in the wild-type background, whereas strong GFP signal is detected in plants carrying a full-length promoter or with the P1 fragment deleted ( Supplementary Fig. 6b ). ChIP using antibodies against histone H3 with different degrees of methylation at its K4 position showed that the P3 and P4 region was significantly enriched in H3K4me3 ( Fig. 3e ). P1, P2 and P6 regions displayed low-degree enrichment, indicating that WOX5 may be under the regulation of multiple transcription factors, other than that of ROW1. The levels of H3K4me3 present in the WOX5 proximal promoter region in both the row1-3 and wox5-1 mutants remained unchanged ( Supplementary Fig. 7 ). A substantial reduction of the total amounts of H3K4me3 in sdg2-1 , a major histone H3 lysine 4 trimethyltransferase in Arabidopsis [33] , is correlated with a significant WOX5 upregulation ( Supplementary Fig. 8 ). A deletion mutant of ROW1 that lacks the 49-amino-acid PHD lost all ability to restore the row1-3 root phenotype as well as its binding to the WOX5 promoter region ( Fig. 3f and Supplementary Fig. 9 ), whereas a 474-amino-acid C-terminal peptide of ROW1 complemented the phenotype ( Fig. 3f ). Despite the fact that ROW1 binds effectively to the DNA fragment 4 of the WUS promoter, the gel shift assay showed it had no significant affinity to any of the DNA fragments of WOX5 promoter used for ChIP assays ( Supplementary Fig. 10 ).These results support the notion that ROW1 binds to histones in the proximal WOX5 promoter region through recognition of H3K4me3 and that a functional PHD is essential for this interaction. 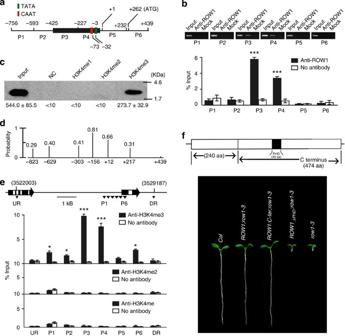Figure 3: ROW1 specifically binds to H3K4me3 in theWOX5promoter region. (a) Schematic diagram showing theWOX5promoter region used in the ChIP assay. (b) ChIP analysis of differentWOX5promoter regions using antibodies against ROW1. Upper panel, RT–PCR analysis. Input, 50 ng genomic DNA obtained from each respective promoter region; anti-ROW1, 10 μg of ROW1-specific antibodies were included in the reaction to precipitate the DNA; mock, negative control with no antibody added. Lower panel, qPCR analysis. Signal intensities were normalized relative to the input and were calculated from three independent experiments. (c) Purified PHD from ROW1 interacted only with biotinylated H3 peptides that were trimethylated at K4. Bound peptides were detected by western blot using biotin antibodies. (d) Theoretical analysis of nucleosome positioning along theWOX5promoter region using a previously reported computational model32. Thexaxis denotesWOX5chromosomal sequence from nucleotide −823 to +439 with the transcription initiation site set to +1. Theyaxis denotes the probability of predicted nucleosomes using the scale of 0.0–1.0. The exact positions of individual base pairs that has a >0.2 probability to initiate a nucleosome are shown as vertical black lines. (e) ChIP analysis of the sameWOX5promoter regions using antibodies against H3K4me3, H3K4me2 or H3K4me. Upper panel, genomic location ofWOX5is shown together with its direction of transcription. DR, downstream region; UR, upstream region. Lower panel, qPCR analysis. Signal intensities were normalized relative to the input and were calculated from three independent reactions. (f) ROW 1 or its C-terminal peptide (C-ter, 474 amino acids) rescued therow1-3phenotype, but a ROW1 construct with a 49-amino-acid deletion of the PHD failed to do so. Shown are 7-day-old seedlings of various genotypes carrying different constructs. Error bars represent s.e. from three biological replicates. *, *** denotesP<0.05 orP<0.001, compared with the negative control with no antibody added, respectively. Uncropped images of panels b and c are shown inSupplementary Fig. 14. Figure 3: ROW1 specifically binds to H3K4me3 in the WOX5 promoter region. ( a ) Schematic diagram showing the WOX5 promoter region used in the ChIP assay. ( b ) ChIP analysis of different WOX5 promoter regions using antibodies against ROW1. Upper panel, RT–PCR analysis. Input, 50 ng genomic DNA obtained from each respective promoter region; anti-ROW1, 10 μg of ROW1-specific antibodies were included in the reaction to precipitate the DNA; mock, negative control with no antibody added. Lower panel, qPCR analysis. Signal intensities were normalized relative to the input and were calculated from three independent experiments. ( c ) Purified PHD from ROW1 interacted only with biotinylated H3 peptides that were trimethylated at K4. Bound peptides were detected by western blot using biotin antibodies. ( d ) Theoretical analysis of nucleosome positioning along the WOX5 promoter region using a previously reported computational model [32] . The x axis denotes WOX5 chromosomal sequence from nucleotide −823 to +439 with the transcription initiation site set to +1. The y axis denotes the probability of predicted nucleosomes using the scale of 0.0–1.0. The exact positions of individual base pairs that has a >0.2 probability to initiate a nucleosome are shown as vertical black lines. ( e ) ChIP analysis of the same WOX5 promoter regions using antibodies against H3K4me3, H3K4me2 or H3K4me. Upper panel, genomic location of WOX5 is shown together with its direction of transcription. DR, downstream region; UR, upstream region. Lower panel, qPCR analysis. Signal intensities were normalized relative to the input and were calculated from three independent reactions. ( f ) ROW 1 or its C-terminal peptide (C-ter, 474 amino acids) rescued the row1-3 phenotype, but a ROW1 construct with a 49-amino-acid deletion of the PHD failed to do so. Shown are 7-day-old seedlings of various genotypes carrying different constructs. Error bars represent s.e. from three biological replicates. *, *** denotes P <0.05 or P <0.001, compared with the negative control with no antibody added, respectively. Uncropped images of panels b and c are shown in Supplementary Fig. 14 . Full size image QC expression of ROW1 represses WOX5 transcription To confirm that ROW1 represses WOX5 expression in vivo , we ectopically expressed ROW1 in the QC using the WOX5 promoter. As a control for the study, ROW1::mCherry-ROW1 was introduced into wild-type Arabidopsis plants expressing the WOX5::GFP construct. As expected, red fluorescenct signal from mCherry was observed only in the PM, not in the QC, whereas green GFP fluorescence was observed strictly in the QC ( Fig. 4a , upper panel). When expressed in row1-3 , the ROW1::mCherry-ROW1 construct was able to complement the mutant phenotype ( Supplementary Fig. 11 ). Only the red fluorescent protein (RFP) signals from mCherry-ROW1 expression were detected from the plants carrying both WOX5::GFP and WOX5::mCherry-ROW1 constructs. Although we expect that ectopic QC expression of mCherry-ROW1 will inhibit the WOX5 promoter activity eventually, we propose that (1) a minimal amount of mCherry-ROW1 has to be present in the QC to repress the WOX5 promoter activity and (2) that mCherry [34] is more stable than the GFP, which originated from Dr5::GFP [35] , and that as a result, only the red mCherry RFP, and not the green GFP signal, was observed in the QC ( Fig. 4a , lower panel). Inhibition of WOX5 expression resulted in a wox5-1 -like DM structure with substantial starch granule accumulation in the DSC layer ( Figs 4b and 2f ), suggesting that the DSCs in these plants underwent premature differentiation as well. This conclusion was verified by a 5-ethynyl-2′-deoxyuridine (EdU) incorporation assay of active cell division [36] . In wild-type Arabidopsis roots, regardless of a WOX5::GFP construct, cell division was observed in both PM and the DSC layer, not in the QC ( Fig. 4c ). However, no EdU incorporation was observed in the cell layer beneath the QC niche in plants expressing the WOX5::mCherry-ROW1 construct ( Fig. 4c ), indicating that QC expression of WOX5 is essential for maintenance of DSC activity. Similar EdU incorporation pattern was observed in either wox5-1 ( Fig. 4c ) or in wox5-1 / row1-3 double mutant ( Supplementary Fig. 12 ) in which the DSC cell layer is known to undergo premature cell differentiation [10] . A regular and well-organized DM structure was found in the roots that expressed WOX5::GFP, whereas a disordered columella cell arrangement was observed in both wox5-1 and wild-type plants expressing the WOX5::GFP and WOX5::mCherry-ROW1 constructs together ( Fig. 4d ). These data indicate that QC expression of ROW1 inhibits WOX5 transcription and results in premature differentiation of the DSCs and disruption of the regular columella cell structure in root tips. Taken together with previous publications [23] , [24] , we suggest that both WUS and WOX5 are negatively regulated by the plant homologue of animal tumour suppressor-like gene ROW1 . 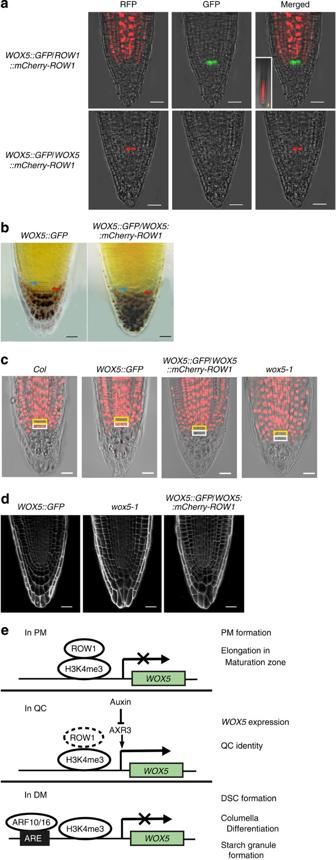Figure 4: QC expression ofROW1reduced the amount ofWOX5transcripts dramatically with a resultant loss of DSC. (a) GFP signals (green) were observed in QC and RFP signals (red) from mCherry-ROW1expression were observed in the PM from plants carrying bothWOX5::GFPandROW1::mCherry-ROW1constructs (upper panel), whereas only the RFP signals from mCherry-ROW1expression were detected from the plants carrying bothWOX5::GFPandWOX5::mCherry-ROW1constructs (lower panel). (b) Root tips ofWOX5::GFPplants showed normal QC (blue arrow) and DSC (red arrow, no starch granule) development, whereas starch granules appeared after staining with Lugol’s solution in the root tips ofWOX5::GFP/WOX5::mCherry-ROW1plants. (c) EdU assay showing normal mitotic activity in wild-type (col) root tip, in root tips of wild-type plants that express theWOX5::GFPconstruct (WOX5::GFP), whereas no such mitotic activity was observed in the same cell layer in plants expressed theWOX5::mCherry-ROW1construct, similar to that ofwox5-1. Yellow box, QC position; The white box below, DSC. (d) Three-dimensional reconstruction showing disrupted columella cell structure in 5-day-old root tips of bothwox5-1andWOX5::GFP/WOX5::mCherry-ROW1. (e) A working model depicts the involvement of ROW1 during development of theArabidopsisroot stem cell niche. Scale bars, 20 μm in this figure. Figure 4: QC expression of ROW1 reduced the amount of WOX5 transcripts dramatically with a resultant loss of DSC. ( a ) GFP signals (green) were observed in QC and RFP signals (red) from mCherry- ROW1 expression were observed in the PM from plants carrying both WOX5::GFP and ROW1::mCherry-ROW1 constructs (upper panel), whereas only the RFP signals from mCherry- ROW1 expression were detected from the plants carrying both WOX5::GFP and WOX5::mCherry-ROW1 constructs (lower panel). ( b ) Root tips of WOX5::GFP plants showed normal QC (blue arrow) and DSC (red arrow, no starch granule) development, whereas starch granules appeared after staining with Lugol’s solution in the root tips of WOX5::GFP/WOX5::mCherry-ROW1 plants. ( c ) EdU assay showing normal mitotic activity in wild-type ( col ) root tip, in root tips of wild-type plants that express the WOX5::GFP construct ( WOX5::GFP ), whereas no such mitotic activity was observed in the same cell layer in plants expressed the WOX5::mCherry-ROW1 construct, similar to that of wox5-1 . Yellow box, QC position; The white box below, DSC. ( d ) Three-dimensional reconstruction showing disrupted columella cell structure in 5-day-old root tips of both wox5-1 and WOX5::GFP/WOX5::mCherry-ROW1 . ( e ) A working model depicts the involvement of ROW1 during development of the Arabidopsis root stem cell niche. Scale bars, 20 μm in this figure. Full size image As depicted in a working model in Fig. 4e , we propose that, in the wild-type Arabidopsis PM zone, ROW1 is bound to the H3K4me3 present on the WOX5 promoter and represses its transcription to allow normal PM cell differentiation and elongation in the maturation zone. However, while we show that ROW1 is able to repress WOX5::GFP when ectopically expressed in the QC, deletion of the proposed ROW1-binding sites in the WOX5 promoter did not induce WOX5 expression in the PM ( Supplementary Fig 6b ). This suggests that the P3 and P4 promoter fragments are also necessary for WOX5 activation and we cannot conclusively exclude the possibility that ROW1-mediated repression of WOX5 in the PM is indirect. In animals, the tumour suppressor protein ING2, which is also a PHD domain-containing protein, represses target gene transcription by binding to H3K4me3 histone markers [21] . In the QC, absence of ROW1 permits the expression of WOX5 and thus maintains the QC identity. Auxin is the only molecule previously known to modulate QC function and distal stem cell differentiation by negatively regulating WOX5 expression [13] , [14] , [15] . Significantly elevated WOX5 expression in cells immediately above the DM in the root tips of row1-3 may potentiate the diffusion of this small polypeptide, as was previously postulated [37] , to nullify ARF10/16 functions that prevented normal DM differentiation. We thus conclude that ROW1 is essential for the development of the whole stem cell niche in Arabidopsis roots by confining WOX5 expression specifically to within the QC. Also, in the wild-type background, WOX5::GFP signals disappeared after 3 days of auxin treatment ( Supplementary Fig. 13a ), whereas no such repression for ROW1::GFP in the wild type and WOX5::GFP in the row1-3 background were observed after the same treatment ( Supplementary Fig. 13b,c ), indicating that ROW1 may regulate WOX5 expression downstream of auxin signalling. ROW1 may be the first reported key repressor that maintains both the SAM [23] , [24] and the root apical meristem identity by interacting with two different master regulators of Arabidopsis stem cell development. Plant lines and growth conditions The Arabidopsis mutant lines with disrupted ROW1 and WOX5 are T-DNA insertion alleles obtained from the SALK collections (Arabidopsis Biological Resource Center, USA; http://signal.salk.edu ): row1-3 , SALK_003498 and wox5-1 , SALK_038262. Seeds were surface sterilized with 0.1% HgCl 2 , germinated on Murashige and Skoog (MS) medium for 2 weeks, transferred to soil and grown in an Intellus control system (Percival) with a 16/8-h light/dark cycle at 22 °C in 70% humidity [38] . For microscopic analyses of gravitropism, seedlings grown in 1/2 MS medium in petri dishes were gravistimulated by rotating the stage 135° for the specified amount of time before imaging. Degrees of bending (mean±s.e.) were calculated from 10 independent main roots of each type. Plant crosses Pollen collected from wox5-1 plants was used to pollinate heterozygous row1-3 plants to produce the homozygous wox5-1/row1-3 double mutant. Transgenic plants carrying WOX5::GFP in the wild-type background [31] were used for crossing with heterozygous row1-3 . Plants that were homozygous for the row1-3 mutation were used to search for the GFP marker in the F2 population. All analyses were performed using seedlings from the F3 generation. The transgenic SCR::GFP line (CS3999) and J0571 line (CS9094) were obtained from the SALK collections. SCR::GFP and J0571 marker lines were crossed to homozygous wox5-1 , heterozygous wox5-1/row1-3 and to heterozygous row1-3 plants. In all analyses, parental lines were used as the controls. Vector construction and plant transformation A ROW1::GFP line was obtained by transforming wild-type Arabidopsis plants with a vector in which the GFP expression was driven by the 1.9-kb ROW1 promoter. The plasmid for WOX5 RNAi was generated by cloning a 367-bp WOX5 fragment from the 3′-transcribed region into the pB7GWIWG2 vector to create a double-stranded WOX5 RNAi cassette driven by the constitutive cauliflower mosaic virus 35S promoter. This construct was then transformed into heterozygous row1-3 plants to produce homozygous seedlings in the next generation. For genetic complementation of the row1-3 phenotype, a 6.1-kb genomic DNA fragment that encompassed the entire ROW1 (At1g04020) coding region plus 1.9 kb of the 5′ upstream sequence and 0.7 kb of downstream flanking sequence was cloned into pCAMBIA1305 using the primers described in Supplementary Table 1 . This construct was then transformed into the heterozygous row1-3 Arabidopsis plants. The fusion ROW1 protein that lacked the PHD (residues 403–451) or C terminus (residues 241–714) was cloned into pCAMBIA3301 that contained the same ROW1 promoter and downstream flanking sequences. Transgenic lines were selected by antibiotic resistance, genomic PCR and also by co-segregation studies that searched for single-copy insertion events into the row1-3 homozygous background. We used 7-day-old seedlings of various genotypes carrying different constructs for phenotype analysis. The mCherry [34] coding sequence was fused in-frame to the ROW1 cDNA, and the resulting fusion was inserted into pQG110 carrying a 4.8 kb WOX5 promoter or the 1.9 kb ROW1 promoter, for transformation into the WOX5::GFP Arabidopsis line. Transgenic Arabidopsis plants were generated by the floral dip method and were selected on solid half-strength MS medium plates containing 50 mg ml −1 of the appropriate antibiotics. RNA extraction and qRT–PCR Root and shoot apices were harvested from 7-day-old wild-type, row1-3 wox5-1 Arabidopsis seedlings. RNA extraction and qRT–PCR were performed as reported [24] . Seedlings (100 mg) were frozen in liquid nitrogen for RNA extraction with the RNeasy mini kit (Qiagen). Complementary DNA was synthesized from 5 μg of total RNA using reverse transcriptase (Fermentas), and the housekeeping gene UBQ5 was used as the internal control. We used triplicate independent plant samples for all PCR analyses with the primers shown in Supplementary Table 1 . We used the CT value method to quantify the relative amount of target gene transcripts as reported [24] . The relative value was calculated by the equation Y =1.8 Δ C t (Δ C t is the differences of C t between the target products and the control UBQ5 products). Statistical significance was evaluated by Student’s t -test. Sequence alignment Multiple sequence alignment was performed using MAFFT [39] and phylogenetic trees were constructed by the neighbour-joining method in MEGA5 (ref. 40 ). Starch staining Arabidopsis roots (7-day old) were dipped in Lugol’s staining solution (Sigma-Aldrich) for 60 min, washed with distilled water and then observed under a differential interference contrast microscope (Leica DMRE). Histological analysis To prepare semi-thin sections, root tips were stained in 1% (w/v) periodic acid solution containing Schiff’s reagent and were fixed overnight in 2% (w/v) paraformaldehyde and 2.5% (w/v) glutaraldehyde in PBS, pH 7.2, at 4 °C. Specimens were then dehydrated in an ethanol series (30, 50, 70, 80, 90, 95 and 100%) and embedded in Spurr’s resin (Spi-Chem). The tissue was mounted in double-distilled H 2 O and sectioned at a thickness of 2 μm on a Leica RM 2265 microtome (Leica). Sections were observed under bright-field optics using a Leica DMRE microscope and cell lengths were measured by SPOT 4.6 Advanced software (Diagnostic Instrument, USA). ChIP assays ChIP was performed as described [41] using 7-day-old plants. For immunoprecipitation, 10 μg of commercial polyclonal antibodies against H3K4me3 (07-473), H3K4me2 (07-030) or H3K4me (07-436, Upstate/Millipore) or 10 μg of ROW1 polyclonal antibody [24] , were incubated in PBS solution with Protein A-agarose, in the presence of 1 mg chromatin extracts. One μg of immunoprecipitated DNA was used for each PCR assay. As negative controls, we performed the ChIP experiments using protein A-agarose without antibody. Relative enrichment of associated DNA fragments was analysed by qPCR. All oligonucleotide sequences used for target DNA detection and quantification in ChIP experiments are shown in Supplementary Table 1 . EdU assay Root tips of germinating Arabidopsis seedlings were submerged in 1 μM EdU in half-strength MS medium for 24 h (ref. 36 ). They were then fixed for 30 min at room temperature in a 4% (w/v) formaldehyde solution in PBS with 0.1% (v/v) Triton-X-100. The fixative was washed away with PBS (three 10-min washes) and the root tip sections were incubated in an EdU detection cocktail (Invitrogen, Click-iT EdU Alexa Fluor 555 Imaging Kit) for 30 min followed by three10-min washes with PBS. The sections were mounted in VECTASHIELD H-1000 anti-fade solution (Vector Laboratories) before being visualized using 545- to 600-nm wavelengths for EdU under an LSM 710 NLO with Duoscan confocal microscope (Zeiss, Germany). Histone peptide-binding assays Biotinylated histone peptides H3K4me1 (12-563), H3K4me2 (12-460) and H3K4me3 (12-564) were bought from Upstate/Millipore, and H3K9me3 and H3K27me3 were provided described previously [42] . For the peptide-binding assay, each peptide (1 μg) was incubated with His-ROW1-PHD bound to Ni-NTA agarose beads in buffer containing 50 mM Tris-HCl, (pH 7.7), 300 mM NaCl and 0.1% (v/v) Nonidet P-40 for 1 h at 4 °C (ref. 20 ). The beads were washed five times for 30 min each in washing buffer at 4 °C, and the samples were separated by 15%Tris-tricine polyacrylamide gel electrophoresis and subjected to western blot analysis with antibody against biotin (Santa Cruz, sc-53179, 1:50) [43] . Confocal microscopy For confocal microscopic analyses, 7-day-old seedlings grown in half-strength MS medium were stained with 10 μg ml −1 propidium iodide for 5 min (ref. 10 ), washed briefly in double-distilled and visualized at 600–640 nm for propidium iodide, 500–560 nm for GFP and 590–630 nm for mCherry RFP on the LSM 710 NLO with Duoscan confocal microscope. For three-dimensional reconstruction of wild type, wox5-01 and WOX5::GFP/WOX5::mCherry-ROW1 root tips, the cell walls were first visualized by staining with 10 μg ml −1 propidium iodide. A series of images was obtained by z -stack scanning and processed by ImarisX64 7.6.04 (Bitplane, Switzerland) to build the three-dimensional structure. How to cite this article: Zhang, Y. et al . ROW1 maintains quiescent centre identity by confining WOX5 expression to specific cells. Nat. Commun. 6:6003 doi: 10.1038/7003 (2015).